Insects with 100 million-year-old dinosaur feathers are not ectoparasites 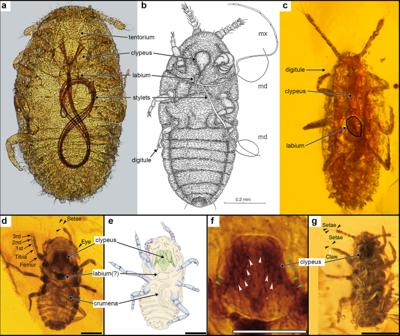Fig. 1: Early instar nymphal Coccoidea, both recent and fossil. Imagesd–gare from the original report by Gao et al. (ref.1).aCrawler of the extant speciesMarchalina hellenica(Margarodidae), ventral view, showing the internal, figure-8 coiled feeding stylets (the crumena) through the translucent body wall. From ref.16, the crumena is commonly a single coil.bEarly instar nymph of pityococcid in Baltic amber (ventral view), from ref.14(original drawing by late Jan Koteja). The feeding styles are fully everted.cEarly instar nymph, family undetermined, in Burmese amber, AMNH Bu-1327. Ventral view, slightly oblique laterally (making nymph appear slightly thinner than actual). Location of the labium is outlined. Stylets are not everted, and crumena not visible through the opaque body wall. Figuresd–g: From Gao et al. (2019, ref.1). The labels outlined in white are ours; all others are original. Permissions:a, ©2006 International Bee Research Association, reprinted by permission of Taylor & Francis Ltd.,http://www.tandfonline.comon behalf of ©2006 International Bee Research Association.b, courtesy of Dr. Paweł Koteja. Further information on research design is available in the Nature Research Reporting Summary linked to this article.